NAA10 controls osteoblast differentiation and bone formation as a feedback regulator of Runx2 Runt-related transcription factor 2 (Runx2) transactivates many genes required for osteoblast differentiation. The role of N -α-acetyltransferase 10 (NAA10, arrest-defective-1), originally identified in yeast, remains poorly understood in mammals. Here we report a new NAA10 function in Runx2-mediated osteogenesis. Runx2 stabilizes NAA10 in osteoblasts during BMP-2-induced differentiation, and NAA10 in turn controls this differentiation by inhibiting Runx2. NAA10 delays bone healing in a rat calvarial defect model and bone development in neonatal mice. Mechanistically, NAA10 acetylates Runx2 at Lys225, and this acetylation inhibits Runx2-driven transcription by interfering with CBFβ binding to Runx2. Our study suggests that NAA10 acts as a guard ensuring balanced osteogenesis by fine-tuning Runx2 signalling in a feedback manner. NAA10 inhibition could be considered a potential strategy for facilitating bone formation. During bone development and regeneration, many transcription factors must be orchestrated to promote osteoblast differentiation. In particular, Runt-related transcription factor 2 (Runx2) leads the differentiation during the early phase. Runx2 requires CBFβ (a non-DNA-binding partner), which allosterically enhances Runx2 binding to DNA [1] , [2] . The Runx2–CBFβ complex binds to a conserved nucleotide sequence (R/TACCRCA), and turns on the expressions of several osteogenic proteins, such as, collagen α1, osteopontin, bone sialoprotein (BSP) and osteocalcin (OCN) [3] , [4] . During osteoblast differentiation, Runx2 is upregulated at the protein level and activated functionally, and these processes are modulated by post-translational modifications of Runx2. Runx2 is activated by being phosphorylated at its serine or threonine residues through the mitogen-activated protein kinase–extracellular signal-regulated kinase pathway, which is stimulated by fibroblast growth factor-2 (refs 5 , 6 ). However, when Runx2 is phosphorylated at other serine residues by GSK3β and CDK4, it becomes destabilized and functionally repressed [7] . Acetylation also modulates the Runx2 signalling pathway. Acetylation at histone lysine residues reorganizes the chromatin structure surrounding Runx2–DNA complexes to induce gene expression [8] , [9] . Furthermore, Runx2 can be lysyl-acetylated directly by some acetyltransferases. For instance, p300 and PCAF (p300/CBP-associated factor) have been reported to acetylate Runx2 at lysine residues and to enhance the transcriptional activity of Runx2 (ref. 10 ). In addition, the acetylation can stabilize Runx2 by inhibiting the Smurf1-mediated ubiquitination of Runx2 (refs 11 , 12 ). Similarly, the acetyltransferases MOZ (monocytic leukaemia zinc finger protein) and MORF (MOZ-related factor) have been reported to activate Runx2, but it remains unclear whether they directly acetylate Runx2 (ref. 13 ). The acetyltransferase arrest-defective-1 (ARD1), which is officially referred to as N -α-acetyltransferase 10 (NAA10), was first identified in Saccharomyces cerevisiae and has been found to be crucial for yeast growth and sporulation [14] . Its orthologs have been identified in mouse and human cells, and participate in cell growth and proliferation, as shown in yeasts [15] . Functionally, NAA10 catalyses the amino-terminal α-acetylation of proteins in yeast and mammalian cells [16] , and it is also known to induce the lysine ε-acetylation of several proteins, including β-catenin, myosin light-chain kinase and androgen receptor [17] , [18] , [19] . Because NAA10 is ubiquitously expressed in many human cells, it is expected to have diverse functions in addition to cell cycle regulation. However, the role of NAA10 remains poorly understood in human cells. In particular, no study has investigated the role of NAA10 in bone formation. In this regard, we investigated the involvement of NAA10 in osteogenesis via the regulation of Runx2 in vitro and in vivo . Our study demonstrates that NAA10 is induced by Runx2 during osteoblast differentiation and in turn controls this differentiation by acetylating and inactivating Runx2. The repair of rat calvarial defects was facilitated by NAA10 knock down and neonatal bone development was delayed in NAA10 transgenic mice. NAA10 may contribute to balanced osteogenesis by fine-tuning Runx2 signalling in a feedback manner, and could be considered a potential target for promoting bone formation. NAA10 negatively regulates osteoblast differentiation To examine the role of NAA10 in bone formation, we analysed NAA10 expression in pre-existing and newly formed bones in rat calvaria with regional bone loss. NAA10 is expressed in osteoblasts around new bone surfaces, whereas it is rarely expressed in pre-existing bones ( Fig. 1a ). In primary mouse osteoblasts and C 2 C 12 cells undergoing BMP-2-induced differentiation, NAA10 is upregulated in parallel with Runx2 induction ( Fig. 1b ; Supplementary Figs 1a and 2 ). Even in the absence of BMP-2, Runx2 and NAA10 levels increase together during the late stage of the culture process ( Fig. 1b , middle). In mouse embryos, both Runx2 and NAA10 are strongly expressed in vertebral bones on embryonic day 13 and their levels decrease gradually later ( Supplementary Fig. 3 ). To examine the role of NAA10 in osteoblast differentiation, markers for osteoblast differentiation, such as alkaline phosphatase (ALP), OCN, BSP and matrix mineralization, were measured. NAA10 acts as an inhibitory player in osteoblast differentiation induced by BMP-2 ( Fig. 1c–e ; Supplementary Fig. 1b–d ). This action of NAA10 is also shown in MC3T3-E1 pre-osteoblast cells treated with BMP-2 ( Supplementary Fig. 4 ). Besides BMP signalling pathways, the Wnt/β-catenin signalling pathway has been reported to play a role in osteoblast differentiation and maturation [20] . Further, NAA10 has been reported to acetylate and activate β-catenin in lung cancer cell lines [17] . In the present study, however, NAA10 does not regulate Wnt3a-stimulated osteoblast differentiation ( Supplementary Fig. 5 ). The role of NAA10 in chondrocyte differentiation was examined because BMP signalling and the subsequent activation of Runx2 are known to promote chondrogenesis [21] . The results indicate that NAA10 is not upregulated in conjunction with Runx2 induction in chondrocytes ( Supplementary Fig. 6a ) and that it is not involved in chondrocyte differentiation ( Supplementary Fig. 6b–d ). NAA10 may be restrictively involved in BMP-2-induced osteoblast differentiation. 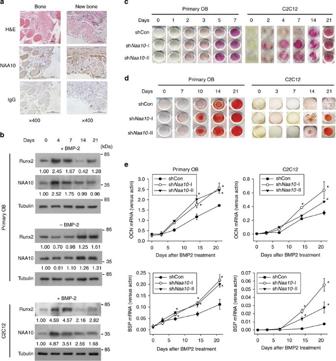Figure 1: NAA10 negatively regulates osteoblast differentiation. (a) A rat calvarial bone was punched out and covered with a collagen sponge containing 1 mg of BMP-2. After 2 months, the bone was removed, fixed, decalcified, paraffin embedded and cut into 5-μm sections. The sections including the margin of defect were stained with H&E or immunostained with anti-NAA10 (scale bar, 100 μm). Arrows indicate NAA10-positive osteoblasts. (b) Primary osteoblasts and C2C12cells were incubated with PBS or BMP-2 (100 ng ml−1) for the indicated times. Protein levels in lysates were analysed by western blotting using the indicated antibodies, and quantified using ImageJ. Runx2 and NAA10 values were divided by tubulin values and the ratios are expressed with respect to those at zero time. (c) Osteoblasts, which had been infected with non-targeting (shCon) or two differentNaa10-targeting (shNaa10) shRNA viruses, were differentiated with BMP-2. ALP was stained with naphthol AS-MX phosphate. (d) Mineralization in differentiating osteoblasts was stained with Alizarin Red S. The results are the representative pictures of three independent experiments. (e) OCN and BSP mRNA levels were quantified in differentiating osteoblasts by RT-qPCR. Results are expressed as the means±s.d. (n=4) and compared statistically using Student’st-test (*P<0.05 versus the shCon group). Figure 1: NAA10 negatively regulates osteoblast differentiation. ( a ) A rat calvarial bone was punched out and covered with a collagen sponge containing 1 mg of BMP-2. After 2 months, the bone was removed, fixed, decalcified, paraffin embedded and cut into 5-μm sections. The sections including the margin of defect were stained with H&E or immunostained with anti-NAA10 (scale bar, 100 μm). Arrows indicate NAA10-positive osteoblasts. ( b ) Primary osteoblasts and C 2 C 12 cells were incubated with PBS or BMP-2 (100 ng ml −1 ) for the indicated times. Protein levels in lysates were analysed by western blotting using the indicated antibodies, and quantified using ImageJ. Runx2 and NAA10 values were divided by tubulin values and the ratios are expressed with respect to those at zero time. ( c ) Osteoblasts, which had been infected with non-targeting (shCon) or two different Naa10 -targeting (shNaa10) shRNA viruses, were differentiated with BMP-2. ALP was stained with naphthol AS-MX phosphate. ( d ) Mineralization in differentiating osteoblasts was stained with Alizarin Red S. The results are the representative pictures of three independent experiments. ( e ) OCN and BSP mRNA levels were quantified in differentiating osteoblasts by RT-qPCR. Results are expressed as the means±s.d. ( n =4) and compared statistically using Student’s t -test (* P <0.05 versus the shCon group). Full size image Runx2 stabilizes NAA10 during osteoblast differentiation As Runx2 and NAA10 are co-induced during osteoblast differentiation, we checked the possibility that they regulate each other. Runx2 is required for the BMP-2 induction of NAA10 ( Fig. 2a ), whereas NAA10 does not affect Runx2 expression ( Supplementary Fig. 7a ). This role of Runx2 in NAA10 expression was confirmed using primary osteoblasts from heterozygous Runx2-knockout mice ( Supplementary Fig. 7b ). Then the mechanism underlying the Runx2 regulation of NAA10 was investigated. Runx2 is not involved in the expression of Naa10 mRNA ( Fig. 2a ; Supplementary Fig. 7c ). To examine whether Runx2 regulates NAA10 protein, we ectopically expressed green fluorescent protein-NAA10 and found that Runx2 upregulates NAA10 at the post-translational level during osteoblast differentiation ( Fig. 2b ). The stability of NAA10 protein was checked by monitoring its level after blocking de novo protein synthesis ( Supplementary Fig. 7d–f ). NAA10 protein is stabilized Runx2 dependently ( Fig. 2c,d ). Compared with those in BMP2-stimulated osteoblasts, ectopic and endogenous NAA10 proteins in unstimuated osteoblasts were induced to a lesser extent by Runx2 overexpression ( Fig. 2b,e ). These results suggest that Runx2 stabilizes NAA10 in concert with some factor(s) activated by BMP-2. Given a previous report demonstrating that IkBα kinase β (IKKβ) phosphorylates NAA10 at Ser209 and by doing so destructs it through the proteasomes [22] , we examined whether IKKβ is involved in the Runx2 regulation of NAA10. IKKβ knock down reversed the NAA10 destabilization by Runx2 knock down ( Fig. 2d ). Furthermore, IKKβ is negatively regulated by Runx2 during osteoblast differentiation ( Fig. 2e ; Supplementary Figs 1a and 8a ). As expected, IKKβ induces the serine phosphorylation of NAA10, which is inhibited by Runx2 ( Fig. 2f ; Supplementary Fig. 8b ). The results suggest that Runx2 stabilizes NAA10 during osteoblast differentiation through its inhibition of IKKβ-mediated phosphorylation and degradation of NAA10. 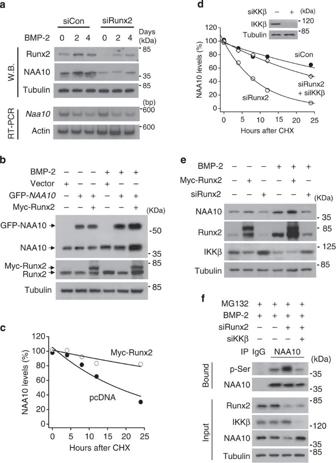Figure 2: NAA10 is stabilized Runx2 dependently during osteoblastogenesis. (a) C2C12cells, which had been transfected with 80 nM siRNA-targetingRunx2, were treated with BMP-2 for 2 or 4 days. Runx2 and NAA10 expressions were analysed by western blotting or semi-quatitative RT-PCR. (b) Primary osteoblasts were cotransfected with the plasmids of green fluorescent protein (GFP)-NAA10(2 μg) and Myc-Runx2 (1 μg) and treated with BMP-2 for 2 days. Protein expressions were analysed by western blotting. (c,d) C2C12cells, which had been transfected with Runx2 siRNA (80 nM) or plasmid (1 μg), were treated with 100 nM cycloheximide for the indicated times. NAA10 and tubulin levels were analysed by western blotting and quantified using ImageJ software. NAA10 values were divided by tubulin values and NAA10/tubulin ratios are expressed with respect to those at zero time. (e) Primary osteoblasts were transfected with the plasmids of Myc-Runx2 or Runx2 siRNA and treated with BMP-2 for 2 days. Expressed proteins were immunoblotted. (f) C2C12cells, which were transfected with Runx2 and/or IKKβ siRNAs, were incubated with BMP-2 for 24 h and further treated with 20 μM MG132 for 8 h. Cell lysates were immunoprecipitated with anti-NAA10, and the precipitates were immunoblotted with phosphoserine (p-Ser) antibody. The input levels of NAA10, Runx2 and IKKβ were verified by western blotting. Figure 2: NAA10 is stabilized Runx2 dependently during osteoblastogenesis. ( a ) C 2 C 12 cells, which had been transfected with 80 nM siRNA-targeting Runx2 , were treated with BMP-2 for 2 or 4 days. Runx2 and NAA10 expressions were analysed by western blotting or semi-quatitative RT-PCR. ( b ) Primary osteoblasts were cotransfected with the plasmids of green fluorescent protein (GFP)- NAA10 (2 μg) and Myc-Runx2 (1 μg) and treated with BMP-2 for 2 days. Protein expressions were analysed by western blotting. ( c , d ) C 2 C 12 cells, which had been transfected with Runx2 siRNA (80 nM) or plasmid (1 μg), were treated with 100 nM cycloheximide for the indicated times. NAA10 and tubulin levels were analysed by western blotting and quantified using ImageJ software. NAA10 values were divided by tubulin values and NAA10/tubulin ratios are expressed with respect to those at zero time. ( e ) Primary osteoblasts were transfected with the plasmids of Myc-Runx2 or Runx2 siRNA and treated with BMP-2 for 2 days. Expressed proteins were immunoblotted. ( f ) C 2 C 12 cells, which were transfected with Runx2 and/or IKKβ siRNAs, were incubated with BMP-2 for 24 h and further treated with 20 μM MG132 for 8 h. Cell lysates were immunoprecipitated with anti-NAA10, and the precipitates were immunoblotted with phosphoserine (p-Ser) antibody. The input levels of NAA10, Runx2 and IKKβ were verified by western blotting. Full size image NAA10 functionally inhibits Runx2 NAA10’s functional control of Runx2 was examined using 6XOSE-luciferase and OG2-luciferase reporters having the Runx2 response element. The Runx2-driven transcription is negatively regulated by NAA10 ( Fig. 3a,b ). Furthermore, BMP-2 stimulates Runx2 binding to the OCN promoter, which is augmented in the absence of NAA10 ( Fig. 3c ). These results suggest the inhibitory role of NAA10 in Runx2-driven gene expression. 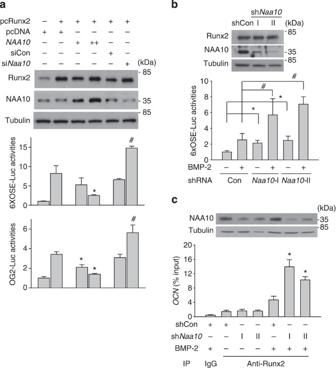Figure 3: NAA10 represses the transcriptional activity of Runx2. (a) C2C12cells were cotransfected with 1 μg of 6XOSE-luciferase plasmid or OG2-luciferase plasmid and β-gal plasmid and with 1 or 2 μg of Runx2 plasmid or 80 nM of Runx2 siRNA. After being allowed to stabilize for 24 h, cells were lysed for western blotting (top) or reporter assays (middle and bottom). Luciferase activities (means+s.d.,n=4) were normalized versus β-gal activity, and are presented as relative values with respect to controls. * and #P<0.05 versus the pcDNA control and versus the siRNA control, respectively. (b) C2C12cell lines infected with shNaa10were cotransfected with 6XOSE-luciferase and β-gal plasmids, and treated with BMP-2 for 24 h. Cells were lysed for western blotting (top) and reporter (bottom) analyses. Luciferase/β-gal values (means+s.d.,n=4) are presented as relative values versus BMP-2 (−) control shRNA. * and #P<0.05 versus BMP-2 (−) control shRNA and versus BMP-2 (+) control shRNA, respectively. (c) C2C12cell lines infected with shNaa10or shControl virus were treated with BMP-2 for 48 h and NAA10 levels were checked by western blotting (top). Cells were then fixed with formalin and cross-linked chromatins were immunoprecipitated with non-immunized serum (IgG) or anti-Runx2. DNAs were eluted from precipitates and real-time PCR was performed to amplify the mouse OCN promoter region. Each bar represents the mean+s.d. (n=4) and *P<0.05 versus the BMP-2 (+) shControl group. Data are statistically analyzed using Student’st-test. Figure 3: NAA10 represses the transcriptional activity of Runx2. ( a ) C 2 C 12 cells were cotransfected with 1 μg of 6XOSE-luciferase plasmid or OG2-luciferase plasmid and β-gal plasmid and with 1 or 2 μg of Runx2 plasmid or 80 nM of Runx2 siRNA. After being allowed to stabilize for 24 h, cells were lysed for western blotting (top) or reporter assays (middle and bottom). Luciferase activities (means+s.d., n =4) were normalized versus β-gal activity, and are presented as relative values with respect to controls. * and # P <0.05 versus the pcDNA control and versus the siRNA control, respectively. ( b ) C 2 C 12 cell lines infected with sh Naa10 were cotransfected with 6XOSE-luciferase and β-gal plasmids, and treated with BMP-2 for 24 h. Cells were lysed for western blotting (top) and reporter (bottom) analyses. Luciferase/β-gal values (means+s.d., n =4) are presented as relative values versus BMP-2 (−) control shRNA. * and # P <0.05 versus BMP-2 (−) control shRNA and versus BMP-2 (+) control shRNA, respectively. ( c ) C 2 C 12 cell lines infected with sh Naa10 or shControl virus were treated with BMP-2 for 48 h and NAA10 levels were checked by western blotting (top). Cells were then fixed with formalin and cross-linked chromatins were immunoprecipitated with non-immunized serum (IgG) or anti-Runx2. DNAs were eluted from precipitates and real-time PCR was performed to amplify the mouse OCN promoter region. Each bar represents the mean+s.d. ( n =4) and * P <0.05 versus the BMP-2 (+) shControl group. Data are statistically analyzed using Student’s t -test. Full size image NAA10 inhibits bone regeneration in adult rats Because injured bone is regenerated through osteoblastogenesis, the role of NAA10 in bone regeneration was examined in a rat calvarial critical-size defect model. Calvarial defects were covered with collagen matrices containing short hairpin RNA (shRNA) viruses and 6 weeks later, the calvarias were examined by microcomputed tomography (CT) to evaluate the extent of bone formation (presented in green). New bone growth occurred inward from margins of calvarial holes covered with BMP-2 matrices, which was substantially augmented by Naa10 shRNA viruses ( Fig. 4a ). We performed the three-dimensional morphometric measurement to analyze the extent to which the calvarial bones healed. Bone regeneration was significantly enhanced by BMP-2 and Naa10 shRNA in combination ( Fig. 4b ). Haematoxylin and eosin (H&E) and von Kossa staining results provided further support the bone regeneration facilitated by NAA10 inhibition ( Fig. 4c ). 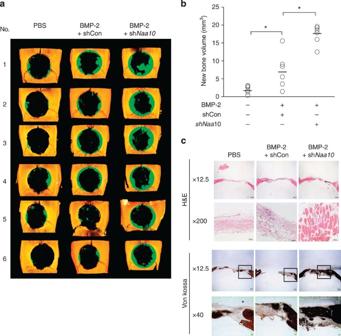Figure 4: NAA10 knock down augments the healing of rat calvarial defects. (a) Six rat calvarial bones per group were punched out and covered with collagen sponge containing BMP-2 (or PBS) and shNaa10virus (or shControl virus). Calvarias were removed on day 42 after surgery and subjected to micro-CT analysis to evaluate defect healing. Micro-CT images were reconstructed three dimensionally; bone ingrowth from defect margins are marked with green. (b) Volumes of ingrown bones were calculated using three-dimensional CT images. Short horizontal bars represent group mean values and *P<0.05 (Student’st-test,n=6) between two groups. (c) Calvarial tissues were fixed, decalcified, embedded and cut into 5-μm sections. The sections were stained with H&E. Calvarial tissues were fixed, embedded and cut into 50-μm sections. The sections were stained with von Kossa/Nuclear Fast Red. The images were captured under a microscope (scale bar, 100 μm). Figure 4: NAA10 knock down augments the healing of rat calvarial defects. ( a ) Six rat calvarial bones per group were punched out and covered with collagen sponge containing BMP-2 (or PBS) and sh Naa10 virus (or shControl virus). Calvarias were removed on day 42 after surgery and subjected to micro-CT analysis to evaluate defect healing. Micro-CT images were reconstructed three dimensionally; bone ingrowth from defect margins are marked with green. ( b ) Volumes of ingrown bones were calculated using three-dimensional CT images. Short horizontal bars represent group mean values and * P <0.05 (Student’s t -test, n =6) between two groups. ( c ) Calvarial tissues were fixed, decalcified, embedded and cut into 5-μm sections. The sections were stained with H&E. Calvarial tissues were fixed, embedded and cut into 50-μm sections. The sections were stained with von Kossa/Nuclear Fast Red. The images were captured under a microscope (scale bar, 100 μm). Full size image NAA10 negatively regulates bone development in mice To understand the role of NAA10 in bone development, the maturation of calvarias during the neonatal stage was examined in wild-type and NAA10 transgenic mice. His/Myc-tagged NAA10 expression vector was used to generate two lines of transgenic mice ( Supplementary Fig. 9 ). Endogenous and transgenic NAA10s were ubiquitously expressed in the skeletons (bones and cartilages) and major organs of transgenic mice ( Supplementary Figs 10 and 11 ). There were no substantial differences in the gross skeletal structures between transgenic mice and wild-type littermates on day 3 after birth ( Supplementary Fig. 15 , left). According to micro-CT analyses, however, calvarial fontanels of NAA10 transgenic mice #10 and #15 were less closed and the bones were less dense, compared with those of their littermates ( Fig. 5a ). Gross morphometric analyses show that calvarial area ( Fig. 5b ) and density ( Fig. 5c ) were significantly reduced in NAA10 transgenic mice. In quantitative micro-CT analyses, the calvarial bones in NAA10 transgenic (#15) mice were identified to be smaller and less dense than those in wild-type mice ( Fig. 5d ). We also examined bone histomorphometry on H&E-stained sections, and found that the osteoblast surface per bone surface is significantly lower in NAA10 transgenic calvaria but the osteoblast number per bone perimeter is not ( Fig. 5e ). In addition, the mRNA levels of the osteoblastogenic genes were substantially reduced in the transgenic calvarias ( Fig. 5f ). These results strongly indicate that bone development is delayed in NAA10 transgenic calvarias because osteoblasts are less active. Femurs were also identified to be less developed in Naa10 transgenic mice on postnatal day 3 ( Supplementary Fig. 12 ). The role of NAA10 in bone development was rechecked using Naa10 -knockout mice. Supplementary Figure 13 shows the Naa10- knockout process and genotyping results. Homozygous Naa10 knock out was verified by checking NAA10 levels in the skeletons and other organs ( Supplementary Fig. 14 ). On day 3 after birth, the skeletal structure appears apparently similar between wild-type and Naa10 -knockout mice, but many bones of knockout mice were more densely stained by Alizarin Red than those of wild-type mice ( Supplementary Fig. 15 , right). In micro-CT images, calvarial ( Fig. 6a–d ) and femoral ( Supplementary Fig. 16 ) bones were developed to a greater extent in Naa10 -knockout mice than in wild-type mice. Osteoblasts in Naa10 -knockout calvarias seem to participate in bone formation more actively ( Fig. 6e,f ). To recheck the inhibitory action of NAA10 on osteoblast differentiation at the cellular level, primary osteoblasts were isolated from the calvarias of wild-type, NAA10 transgenic and Naa10 -knockout mice. As expected, BMP-2-induced osteoblast differentiation is negatively regulated by NAA10 ( Supplementary Fig. 17 ). Taken together, these results strongly indicate the negative role of NAA10 in bone development. 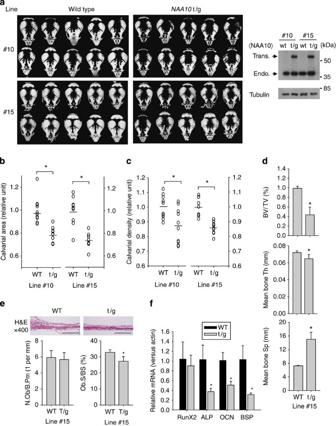Figure 5: Calvarial bone development is delayed inNAA10transgenic mice. (a) Micro-CT images of calvarias were taken from two lines (#10 and #15) ofNAA10transgenic mice and their littermate mice at postnatal 3 day. In each line, 10 transgenic mice and 10 littermate mice were examined. All images were captured at the same magnification, and the representative images are shown. Expression of endogenous and ectopicNAA10in calvarias ofNAA10transgenic mouse line #10 and #15 and their littermates. The lysates were isolated from calvaria and analysed using immunoblotting with anti-NAA10 and β-tubulin (right panel). (b,c) Calvaria area and bone density were analysed in wild-type andNAA10transgenic mice using ImageJ densitometry programme. Short horizontal bars represent group mean values (n=10). (d) Calvarial bone parameters, such as bone volume per tissue volume (BV/TV), mean bone thickness (Th) and mean bone separation (Sp), were analysed from reconstructed three-dimensional images on micro-CT. Results are presented as the means+s.d. (n=5). (e) Calvarias were removed fromNAA10(line #15) transgenic mice and their wild-type littermates on postnatal day 3. Bone tissues were decalcified with EDTA and embedded in paraffin. The calvarial sections (5 μm thickness) were stained with H&E. Representative findings are presented in the top panel (scale bar, 100 μm). Bone formation parameters, such as number of osteoblasts per bone perimeter (N.Ob/B.Pm) and osteoblast surface per bone surface (Ob.S/BS), were analysed using the OsteoMeasure software system (OsteoMetrics, Decatur, GA) and presented as the means+s.d. (n=5). (f) RNAs were extracted from mouse calvarias, and Runx2, ALP, OCN and BSP mRNA levels were quantified by RT–qPCR. Each bar represents the mean+s.d. from six independent samples. *P<0.05 (Student’st-test) versus the corresponding value in the WT group. Figure 5: Calvarial bone development is delayed in NAA10 transgenic mice. ( a ) Micro-CT images of calvarias were taken from two lines (#10 and #15) of NAA10 transgenic mice and their littermate mice at postnatal 3 day. In each line, 10 transgenic mice and 10 littermate mice were examined. All images were captured at the same magnification, and the representative images are shown. Expression of endogenous and ectopic NAA10 in calvarias of NAA10 transgenic mouse line #10 and #15 and their littermates. The lysates were isolated from calvaria and analysed using immunoblotting with anti-NAA10 and β-tubulin (right panel). ( b , c ) Calvaria area and bone density were analysed in wild-type and NAA10 transgenic mice using ImageJ densitometry programme. Short horizontal bars represent group mean values ( n =10). ( d ) Calvarial bone parameters, such as bone volume per tissue volume (BV/TV), mean bone thickness (Th) and mean bone separation (Sp), were analysed from reconstructed three-dimensional images on micro-CT. Results are presented as the means+s.d. ( n =5). ( e ) Calvarias were removed from NAA10 (line #15) transgenic mice and their wild-type littermates on postnatal day 3. Bone tissues were decalcified with EDTA and embedded in paraffin. The calvarial sections (5 μm thickness) were stained with H&E. Representative findings are presented in the top panel (scale bar, 100 μm). Bone formation parameters, such as number of osteoblasts per bone perimeter (N.Ob/B.Pm) and osteoblast surface per bone surface (Ob.S/BS), were analysed using the OsteoMeasure software system (OsteoMetrics, Decatur, GA) and presented as the means+s.d. ( n =5). ( f ) RNAs were extracted from mouse calvarias, and Runx2, ALP, OCN and BSP mRNA levels were quantified by RT–qPCR. Each bar represents the mean+s.d. from six independent samples. * P <0.05 (Student’s t -test) versus the corresponding value in the WT group. 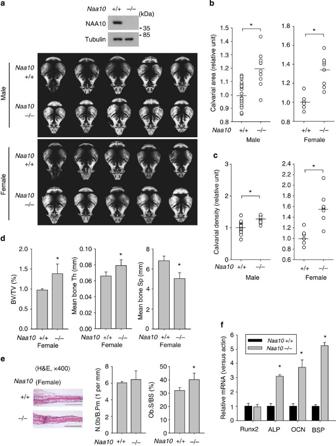Figure 6: Calvarial bone development is facilitated inNaa10−/−-knockout mice. (a) Micro-CT images of calvarias were taken fromNaa10+/+(wt) andNaa10−/−mouse on postnatal day 3. All images were captured at the same magnification, and the representative images are shown. Male and female groups were separately analysed. NAA10 and β-tubulin levels were analysed in the calvarias ofNaa10+/+andNaa10−/−mice by western blotting (right panel). (b,c) Calvarial area and bone density inNaa10+/+andNaa10−/−mice were analysed using ImageJ densitometry programme. Short horizontal bars represent group mean values and *P<0.05 between two groups. Experimental numbers are 24 forNaa10+/+males, 10 forNaa10−/−males, 6 forNaa10+/+females and 8 forNaa10−/−females. (d) Bone parameters, such as BV/TV, mean bone Th and mean bone Sp, were analysed from three-dimensional micro-CT images of calvarias fromNaa10+/+andNaa10−/−female mice (means+s.d.,n=5). (e) Calvarial sections were prepared fromNaa10+/+andNaa10−/−female mice on postnatal day 3 and stained with H&E. Representative findings are presented in the left panel (scale bar, 100 μm). The bone parameters N.Ob/B.Pm and Ob.S/BS were analysed using the OsteoMeasure software and presented as the means+s.d. (n=5). (f) Runx2, ALP, OCN and BSP mRNA levels (means+s.d.,n=6) in mouse calvarias were quantified by RT-qPCR. *P<0.05 versus the corresponding value in the WT group. Data are statistically analysed using Student’st-test. Full size image Figure 6: Calvarial bone development is facilitated in Naa10 −/− -knockout mice. ( a ) Micro-CT images of calvarias were taken from Naa10 +/+ (wt) and Naa10 −/− mouse on postnatal day 3. All images were captured at the same magnification, and the representative images are shown. Male and female groups were separately analysed. NAA10 and β-tubulin levels were analysed in the calvarias of Naa10 +/+ and Naa10 −/− mice by western blotting (right panel). ( b , c ) Calvarial area and bone density in Naa10 +/+ and Naa10 −/− mice were analysed using ImageJ densitometry programme. Short horizontal bars represent group mean values and * P <0.05 between two groups. Experimental numbers are 24 for Naa10 +/+ males, 10 for Naa10 −/− males, 6 for Naa10 +/+ females and 8 for Naa10 −/− females. ( d ) Bone parameters, such as BV/TV, mean bone Th and mean bone Sp, were analysed from three-dimensional micro-CT images of calvarias from Naa10 +/+ and Naa10 −/− female mice (means+s.d., n =5). ( e ) Calvarial sections were prepared from Naa10 +/+ and Naa10 −/− female mice on postnatal day 3 and stained with H&E. Representative findings are presented in the left panel (scale bar, 100 μm). The bone parameters N.Ob/B.Pm and Ob.S/BS were analysed using the OsteoMeasure software and presented as the means+s.d. ( n =5). ( f ) Runx2, ALP, OCN and BSP mRNA levels (means+s.d., n =6) in mouse calvarias were quantified by RT-qPCR. * P <0.05 versus the corresponding value in the WT group. Data are statistically analysed using Student’s t -test. Full size image NAA10 binds to and acetylates Runx2 Next, we addressed the molecular action of NAA10 in the Runx2 signalling pathway. NAA10 physically interacts with Runx2 in differentiating osteoblasts ( Fig. 7a ). This interaction also occurred between NAA10 and Myc-Runx2 expressed in HEK293T cells ( Supplementary Fig. 18a ). Since NAA10 can acetylate the ε-amino group of lysines, it was examined whether NAA10 lysyl-acetylates Runx2. Runx2 under BMP-2 stimulation is basally lysyl acetylated in osteoblasts and this acetylation occurs NAA10 dependently ( Fig. 7b,c ; Supplementary Figs 18b and 19 ). To indentify the Runx2 domain targeted by NAA10, one of the four Flag/SBP-tagged Runx2 fragments (NT, N terminus; RD, RUNT domain; PD, PST domain; CT, C terminus) were coexpressed with NAA10 in HEK293T cells, and then pulled down using Streptoavidin-affinity resins. Of these fragments, RD peptide not only coprecipitated with NAA10 but was also acetylated by NAA10 ( Fig. 7d ), suggesting that NAA10 binds and acetylates the RUNT domain of Runx2. Although Runx2 is localized to the nucleus in osteoblasts, NAA10 is present mainly in the cytoplasm, where it interacts with Runx2 ( Supplementary Fig. 18c,d ). These results suggest that Runx2 is targeted by NAA10 in the cytoplasm before it enters into the nucleus or while it shuttles between the nucleus and the cytoplasm [23] . To identify the entity responsible for the reversal of the NAA10-mediated acetylation of the RUNT domain, we searched for the deacetylase among HDAC members. Of the six HDACs tested, HDAC6 blocks the NAA10-dependent RUNT acetylation ( Fig. 7e ). Given that HDAC6 is expressed at a constant level during osteoblast differentiation ( Supplementary Fig. 1a ), the regulation of Runx2 acetylation is considered to be determined more by NAA10 than by HDAC6. 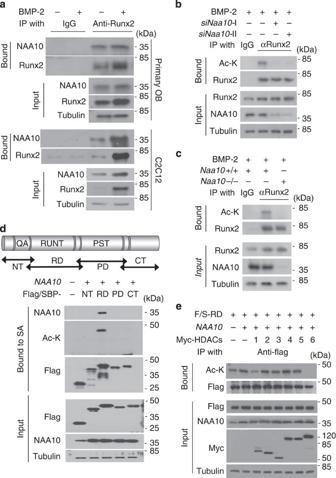Figure 7: NAA10 binds and acetylates the RUNT domain of Runx2. (a) Primary osteoblast cells and C2C12cells were treated with BMP-2 at 100 ng ml−1for 4 days. Cell extracts were then immunoprecipitated with anti-Runx2, and precipitated Runx2 and NAA10 were immunoblotted with specific antibodies. (b) Primary osteoblast cells were transfected withNaa10-targeted siRNAs and treated with BMP-2 at 100 ng ml−1for 4 days. Later, the cells were incubated with 1 μM Trichostatin A (a deacetylase inhibitor) for 6 h. Cell extracts were then immunoprecipitated with anti-Runx2, and its acetylation was analysed by western blotting using an anti-acetyl lysine antibody. (c) Primary osteoblasts from wild-type andNaa10-knockout mice were treated with BMP-2 for 4 days. After being incubated with 1 μM Trichostatin A for 6 h, cells were subjected to immunoprecipitation with anti-Runx2, and Runx2 acetylation was analysed using anti-acetyl lysine antibody. (d) Flag/SBP-tagged Runx2 constructs are illustrated in the top panel. HEK293T cells were cotransfected with plasmids of a Runx2 peptide andNAA10, and treated with Trichostatin A for 6 h. Flag/SBP-peptides were pulled down with streptoavidin-affinity beads and NAA10 coprecipitation and lysyl acetylation were analysed by western blotting. (e) HEK293T cells were cotransfected with plasmids of Flag/SBP-RD,NAA10and Myc-HDACs, and then treated with Trichostatin A for 6 h. Flag/SBP-RD peptide was pulled down using Flag-affinity beads, and the lysyl acetylation of RD peptide was analysed by western blotting. Figure 7: NAA10 binds and acetylates the RUNT domain of Runx2. ( a ) Primary osteoblast cells and C 2 C 12 cells were treated with BMP-2 at 100 ng ml −1 for 4 days. Cell extracts were then immunoprecipitated with anti-Runx2, and precipitated Runx2 and NAA10 were immunoblotted with specific antibodies. ( b ) Primary osteoblast cells were transfected with Naa10- targeted siRNAs and treated with BMP-2 at 100 ng ml −1 for 4 days. Later, the cells were incubated with 1 μM Trichostatin A (a deacetylase inhibitor) for 6 h. Cell extracts were then immunoprecipitated with anti-Runx2, and its acetylation was analysed by western blotting using an anti-acetyl lysine antibody. ( c ) Primary osteoblasts from wild-type and Naa10 -knockout mice were treated with BMP-2 for 4 days. After being incubated with 1 μM Trichostatin A for 6 h, cells were subjected to immunoprecipitation with anti-Runx2, and Runx2 acetylation was analysed using anti-acetyl lysine antibody. ( d ) Flag/SBP-tagged Runx2 constructs are illustrated in the top panel. HEK293T cells were cotransfected with plasmids of a Runx2 peptide and NAA10 , and treated with Trichostatin A for 6 h. Flag/SBP-peptides were pulled down with streptoavidin-affinity beads and NAA10 coprecipitation and lysyl acetylation were analysed by western blotting. ( e ) HEK293T cells were cotransfected with plasmids of Flag/SBP-RD, NAA10 and Myc-HDACs, and then treated with Trichostatin A for 6 h. Flag/SBP-RD peptide was pulled down using Flag-affinity beads, and the lysyl acetylation of RD peptide was analysed by western blotting. Full size image NAA10 inactivates Runx2 by acetylating K225 in RUNT domain To seek for acetylated residues of the RUNT domain, the RUNT peptide was purified in two steps and subjected to liquid chromatography/MASS spectrometry ( Supplementary Fig. 20a ). K183 and K225 of Runx2 are identified to be acetylated ( Supplementary Fig. 20b,c ). A BLAST search (NCBI) revealed that both lysine residues are conserved in various species ( Fig. 8a ). To identify the lysine residue targeted by NAA10, we examined whether RUNT peptide and its mutants (K183R and K225R) were acetylated NAA10 dependently. The K225 residue in Runx2 is a specific site acetylated by NAA10, which was identified in three different experimental settings ( Fig. 8b ; Supplementary Figs 21 and 22 ). To confirm the Runx2 acetylation at K225, an antibody recognizing this modification was generated using a synthetic peptide containing acetylated K225 ( Supplementary Fig. 23a ). The antibody could detect the ARD1-dependent acetylation of K225 in RUNT peptide ( Supplementary Fig. 23b ) and in full-length Runx2 ( Supplementary Fig. 23c ), but not in K225R-mutated Runx2 ( Supplementary Fig. 23d ). The reactivity of the antibody was blocked only by the K225-acetylated peptide, further supporting the antibody specificity to acetylation. By using this antibody, it was successfully demonstrated that endogenous Runx2 is acetylated at K225 depending on NAA10 ( Supplementary Fig. 24e ). Next, we functionally checked the effect of the lysyl acetylation on Runx2-driven transcription, and found that the NAA10-dependent K225 acetylation in Runx2 demotes the Runx2-driven transcription ( Fig. 8c ). In addition, the K225 acetylation disturbs the Runx2 binding to the OCN gene ( Fig. 8d ). As for the mechanism underlying the Runx2 inactivation by NAA10, we thought of the possibility that NAA10 dissociates CBFβ from Runx2 because the transcription coactivator CBFβ interacts with the RUNT domain as NAA10 does. Our results suggest that NAA10 interferes with CBFβ binding to Runx2 by acetylating Runx2 at K225 ( Fig. 9a–c ). 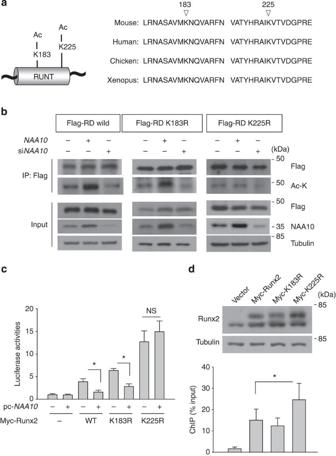Figure 8: NAA10 inhibits the transcriptional activity of Runx2 by acetylating it at K225. (a) Lysine residues 183 and 225 are well conserved among different species. (b) Flag/SBP-RD, Flag/SBP-RD K183R or Flag/SBP-RD K225R plasmids were cotransfected withNAA10plasmid or siRNA into HEK293T cells. After treated with 1 μM Trichostatin A, cells were lysed and incubated with anti-Flag and Flag/SBP-RD peptides and their lysyl acetylations were analysed by western blotting. (c) C2C12cells were cotransfected with OG2-luciferase, β-gal, a Myc-Runx2 (full-length), Myc-Runx2 K183R and Myc-Runx2 K225R plasmids. Luciferase activities (means+s.d.,n=4) were normalized versus β-gal activities and are presented relative to NAA10(−) and Runx2(−) values. (d) C2C12cells, which had been transfected with one of the indicated plasmids, were treated with BMP-2 for 48 h and Runx2 levels were checked by western blotting (top). Cells were fixed with formalin and cross-linked chromatins were immunoprecipitated with anti-Runx2. DNAs were eluted and real-time PCR was performed to amplify the mouse OCN promoter region. *P<0.05 (Student’st-test) between two groups. Figure 8: NAA10 inhibits the transcriptional activity of Runx2 by acetylating it at K225. ( a ) Lysine residues 183 and 225 are well conserved among different species. ( b ) Flag/SBP-RD, Flag/SBP-RD K183R or Flag/SBP-RD K225R plasmids were cotransfected with NAA10 plasmid or siRNA into HEK293T cells. After treated with 1 μM Trichostatin A, cells were lysed and incubated with anti-Flag and Flag/SBP-RD peptides and their lysyl acetylations were analysed by western blotting. ( c ) C 2 C 12 cells were cotransfected with OG2-luciferase, β-gal, a Myc-Runx2 (full-length), Myc-Runx2 K183R and Myc-Runx2 K225R plasmids. Luciferase activities (means+s.d., n =4) were normalized versus β-gal activities and are presented relative to NAA10(−) and Runx2(−) values. ( d ) C 2 C 12 cells, which had been transfected with one of the indicated plasmids, were treated with BMP-2 for 48 h and Runx2 levels were checked by western blotting (top). Cells were fixed with formalin and cross-linked chromatins were immunoprecipitated with anti-Runx2. DNAs were eluted and real-time PCR was performed to amplify the mouse OCN promoter region. * P <0.05 (Student’s t -test) between two groups. 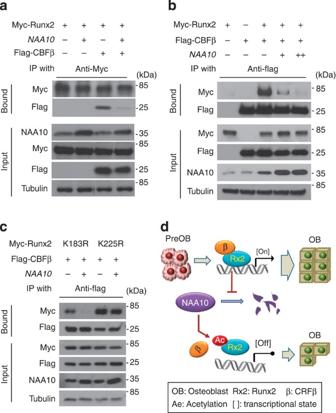Figure 9: NAA10 blocks the Runx2–CBFβ interaction by acetylating Runx2 at K225. (a) HEK293T cells were cotransfected with Myc-Runx2, NAA10 and Flag-CBFβ plasmids. Myc-Runx2 was precipitated with anti-Myc, and coprecipitated Flag-CBFβwas analysed using anti-Flag. (b) In HEK293 cells transfected with 2 or 4 μg ofNAA10, Flag-CBFβ precipitated with anti-Flag and coprecipitated Myc-Runx2 was analysed using anti-Myc. (c) In HEK293 cells transfected with Myc-Runx2 K183R or Myc-Runx2 K225R plasmid, Flag-CBFβ was precipitated with anti-Flag and coprecipitated Myc-Runx2 mutants were analysed using anti-Myc. (d) Proposed mechanism for the role of NAA10 in Runx2-mediated osteoblast differentiation. Full size image Figure 9: NAA10 blocks the Runx2–CBFβ interaction by acetylating Runx2 at K225. ( a ) HEK293T cells were cotransfected with Myc-Runx2, NAA10 and Flag-CBFβ plasmids. Myc-Runx2 was precipitated with anti-Myc, and coprecipitated Flag-CBFβwas analysed using anti-Flag. ( b ) In HEK293 cells transfected with 2 or 4 μg of NAA10 , Flag-CBFβ precipitated with anti-Flag and coprecipitated Myc-Runx2 was analysed using anti-Myc. ( c ) In HEK293 cells transfected with Myc-Runx2 K183R or Myc-Runx2 K225R plasmid, Flag-CBFβ was precipitated with anti-Flag and coprecipitated Myc-Runx2 mutants were analysed using anti-Myc. ( d ) Proposed mechanism for the role of NAA10 in Runx2-mediated osteoblast differentiation. Full size image Runx2 promotes osteoblast differentiation in concert with other osteogenic factors, and thus, its activity should be fine tuned. Given our results, NAA10 functions to ensure the balanced action of Runx2 during osteoblast differentiation. NAA10 is stabilized by Runx2 induced by BMP-2. In turn, NAA10 acetylates Runx2 at Lys225, which disturbs the dimerization of Runx2 and CBFβ and leads to the repression of Runx2-driven transcription. Accordingly, NAA10 checks BMP-2-induced osteoblast differentiation as a feedback regulator of Runx2. The role of NAA10 is summarized in Fig. 9d . Furthermore, based on this scenario, we successfully facilitated bone formation in rat and mouse calvarias by targeting NAA10. Since Naa10 was originally found in yeast cells [14] , [24] , its orthologs have been identified in most mammalian species. However, their functions have not been well defined. NAA10 is known to promote cell proliferation in human lung cancer by activating β-catenin [17] , to control cell migration in human fibrosarcoma by inactivating myosin light-chain kinase [18] , to control neuronal differentiation in mouse brain [25] , [26] and to promote prosate tumorigenesis by facilitating the androgen receptor signalling pathway [19] . However, NAA10 is generally believed (based on its ubiquitous expression) to have additional, as yet unknown, functions in mammalian cells. In the present study, we propose a new function of NAA10 in bone formation. Cellular components of the skeleton, such as, osteoblasts, chondrocytes and myoblasts, are derived from mesenchymal stem cells, whose fates are determined by key transcription factors. The Runx2, Osterix and canonical Wnt signalling pathways drive the differentiation of mesenchymal cells towards the osteoblast lineage [27] . Moreover, spatial and temporal interplay between these factors ensures that the differentiation proceeds to the immature osteoblast stage. However, later osteoblast maturation is not driven by these factors. For example, Runx2 transgenic mice have been found to show severe osteopenia with multiple fractures and depressed OCN in osteoblasts [28] . These findings suggest that Runx2 suppresses osteoblast maturation during the late differentiation stage. In the present study, NAA10 inhibition was found to augment osteoblast differentiation by activating Runx2. In view of the inhibitory effect of Runx2 during the mature osteoblast stage, it appears that NAA10 inhibition could accelerate osteoblast differentiation but delay osteoblast maturation. However, our results regarding OCN, BSP, mineralization and in vivo bone formation showed that NAA10 inhibition can facilitate osteoblast maturation. NAA10 may also be involved in osteoblast maturation. In general, NAA10 is known as the catalytic subunit of NatA that acetylates the α-amino group in nascent peptides [29] . In the NatA complex, NAA10 is heterodimerized with the auxiliary subunit NAA15. A growing body of evidence has suggested that NAA10 has diverse functions beyond the cotranslational modification. NAA10 can catalyse amino-terminal α-acetylation or lysine ε-acetylation in many proteins as post-translational modification [17] , [18] , [19] , [30] , and our results provide additional support for this role of NAA10. Moreover, given our result showing that recombinant NAA10 catalyses lysyl acetylation without auxiliary partners, NAA10 is likely to have its enzymatic activity as a monomer. However, a previous study has demonstrated that NAA15, in association with Ku70 and Ku80, promotes the Runx2-driven transcription of the OCN gene in osteoblasts [31] . Therefore, we examined whether NAA15 is involved in the NAA10 regulation of Runx2, but found that NAA15 is not required for such an action of NAA10 ( Supplementary Fig. 24a–d ). In addition, the acetylation of endogenous Runx2 at K225 was not affected by NAA15 knock down ( Supplementary Fig. 24e ). NAA10 seems to be a solo player that controls osteoblast differentiation by acetylating Runx2 at K225. During the early stage of osteoblast differentiation, Runx2 and NAA10 are induced, whereas IKKβ is downregulated. Moreover, Runx2 induces NAA10 by inhibiting the IKKβ-mediated destabilization of NAA10. Under inflammatory conditions, IKKβ phosphorylates and destabilizes IκBα, which in turn allows NF-κB to enter into the nucleus and thereby to express a variety of proinflammatory genes. Likewise, IKKβ has been known to phosphorylate many proteins other than IκBα and subsequently to inhibit their functions. For instance, the substrates of IKKβ include IRS1, DOK1, FOXO3a and TSC1. Recently, NAA10 was also demonstrated to be destabilized through IKKβ-meidated phosphorylation [22] , and we here found that Runx2 suppresses this action of IKKβ in differentiating osteoblasts. However, how Runx2 downregulates IKKβ is an open question. Given that Runx2 is a transcription factor, we can speculate that Runx2 promotes the expression of IKKβ-degrading proteins such as Keap1 or that it acts as a repressor of the IKKβ gene [32] . Many lines of evidence suggest that Runx2 recruits histone acetyltransferases, such as, CBP, p300, P/CAF, MOZ and MORF, on its target genes. Usually, histone acetyltransferases disentangle tight chromatins and help Runx2 access to DNA, thereby facilitating Runx2-driven transcription [33] . Furthermore, p300 has been reported to stabilize and activate Runx2 by directly acetylating Runx2 (ref. 10 ). A mutational analysis suggested that mouse Runx2 is acetylated at multiple residues including K225, K230, K350 and K351. However, it was not investigated how Runx2 activity is regulated by being acetylated at each lysine residue. In the present study, NAA10 was found to acetylate only K225 of mouse Runx2 and to repress the transcriptional function of Runx2. Consequently, it appears that p300 and NAA10 acetylate Runx2 but regulate Runx2 activity in the opposite manner. The functional consequence of Runx2 acetylation may depend on which residue is acetylated. On the basis of the aforementioned findings, the following scenario can be conceived: with the constant expression of p300, it supports Runx2 activation during the initial stages of osteoblast differentiation. After NAA10 is induced by Runx2, p300 is overwhelmed by NAA10, which then controls Runx2 during the next step in the differentiation process. Future research should test this hypothesis. Core-binding factor β (CBFβ) is a coactivator essential for the activation of Runx proteins (Runx1-3). Although it does not bind to DNA directly, CBFβ enhances the DNA binding of Runx proteins, and thereby, facilitates Runx-driven transcription [34] . Indeed, it has been demonstrated that CBFβ is required for Runx2-dependent bone development during the embryonic and postnatal stages [35] , [36] . In the present study, we found that the NAA10-mediated K225 acetylation of Runx2 blocks CBFβ binding to Runx2. This acetylation may change the confirmation of RUNT domain to a form unfavourable to CBFβ binding. Given the role of CBFβsuggested previously, the dissociation of CBFβ from acetylated Runx2 reasonably explains why NAA10 reduces the DNA binding ability of Runx2. However, as the Runt domain also directly binds to DNA, it is also possible that the acetyl moiety carries a negative charge, and thus, RUNT acetylation repels DNA from Runx2. However, this possibility also remains to be investigated. BMPs are a subfamily of the transforming growth factor-β superfamily and can be divided into several subgroups by sequence homology. BMPs are secreted by osteoblasts and chondrocytes and stimulate their differentiations. Furthermore, BMPs bind to serine/threonine kinase receptors in progenitor cells and induce the phosphorylations of Smads, which enter the nucleus and express skeletogenic genes and other transcription factors [37] , [38] . On the basis of these actions of BMPs, recombinant human BMP-2 and BMP-7 have been clinically tested to promote bone healing in open fractures. The clinical use of collagen matrices containing BMPs has been approved by the U.S. Food and Drug Administration [39] . A number of prospective studies have shown that the implantation of recombinant BMP-2 or BMP-7 significantly increases the union rate and reduces the union time [40] , [41] . In the present study, we covered calvarial defects with a BMP-2 containing collagen, which facilitated bone regeneration. Furthermore, a NAA10-silencing virus augmented the BMP-2-induced bone regeneration. This suggests that NAA10 inhibition in conjunction with BMP-2 treatment offers a potential means for improving fracture healing. Summarizing, this study shows that Runx2 stabilizes NAA10, which in turn inhibits Runx2. This negative feedback loop evidently fine tunes the Runx2 signalling pathway and maintains the balance between Runx2 and other osteogenic factors. For the early rehabilitation of patients with open fracture, early fracture healing is first considered, and thus, it is necessary to investigate the way to accelerate bone regeneration. On the basis of our results, NAA10 inhibition could be considered as one of potential strategies for facilitating fracture healing. Reagents and antibodies Culture media were purchased from Invitrogen (Carlsbad, CA), and fetal calf serum from Sigma-Aldrich (St Louis, MO. Recombinant human BMP-2 (bone morphogenic protein 2) was purchased from Perprotech (Rocky Hill, NJ). A polyclonal antibody against NAA10 was raised in rats against full-length human NAA10 (ref. 17 ). Mouse NAA10 and β-tubulin primary antibodies and horseradish peroxidase-conjugated secondary antibodies were purchased from Santa Cruz Biotechnology (Santa Cruz, CA); anti-Runx2 from MBL (Nagoya, Japan); Acetylated-Lysine antibody from Cell Signaling Technologies (Billerical, MA); anti-α-Myc-tag and Flag-tag antibody from Sigma-Aldrich. Preparation and transfection of plasmids or siRNAs Myc-tagged mouse Runx2 plasmid and 6xOSE/OG2 reporter plasmids were provided by Dr Hyun-Mo Ryoo (Seoul National University School of Dentistry). Human CBFβ cDNA was cloned using reverse transcriptase-PCR (RT-PCR) and inserted into the Myc-tagged pcDNA. The plasmids for Flag/SBP-tagged Runx2 fragments were re-cloned from the mouse Runx2 plasmid using PCR and blunt-end ligation. Site-specific mutations of Runx2 were performed using PCR-based mutagenesis (Stratagene; Cedar Creek, TX). The NAA10 plasmid was constructed as previously described [17] . For transient transfection with plasmids or siRNAs, cells at ~40% density were transfected with plasmids or siRNAs using calcium phosphate or Lipofectamine reagent (Invitrogen). The transfected cells were allowed to be stabilized for 48 h before being used in experiments. The shRNAs containing a hairpin loop were synthesized and inserted into pLKO.1-puro vector. The viral vectors were cotransfected into HEK293T cells with pRSV-Rev, pMD2-VSVG and pMDLg/pRRE plasmids to prepare viral particles. On the third day after transfection, Lenti viruses were collected from the supernatant of HEK293T cells. C 2 C 12 cells were infected with viruses (100 μl ml −1 ) and selected using puromycin (2 μg ml −1 ) to establish stable cell lines. The sequences of siRNAs used are 5′-CCAACACCCTCAACTTTCAGATCAG-3′ for silencing mouse Naa10 and 5′-AUGAACGUGAAUUGCUCAATT-3′ for non-targeting control. The sequences of Naa10 shRNAs are 5′-CCGGCCGGAGAACTACCAGATGAAGCTCGAGCTTCATCTGGTAGTTCTCCGGTTTTT-3′ for mouse sh Naa10 -I, 5′-CCGGACACCCTCAACTTTCAGATCACTCGAGTGATCTGAAAGTTGAGGGTGTTTTTT-3′ for mouse sh Naa10 -II and rat shNAA10, and 5′-CCGGTACAACAGCCACAACGTCTATCTCGAGATAGACGTTGTGGCTGTTGTATTTTT-3′ for non-targeting shRNA. Isolation and culture of mouse primary osteoblasts Calvarias of newborn mice were washed in HBSS (Life Technologies, NY) containing 3% penicillin and streptomycin. Isolated calvarias were sequentially digested in α-MEM containing 0.1% collagenase (Sigma-Aldrich) and 0.2% Dispase II (Roche, Switzerland) at 37 °C. Digestion was carried out five times (for 30 min per each digestion), and the fractions were pooled. Osteoblasts were collected by centrifugation and resuspended in ascorbic acid-free α-MEM. Osteoblasts were plated onto 100-mm culture dishes and the media were replaced 24 h later. To induce differentiation, cells were treated with ascorbic acid (50 μg ml −1 ), β-glycerophosphate (2 mM) and BMP-2 (100 ng ml −1 ). This procedure was approved by the Institutional Animal Care and Use Committee of Seoul National University (Approve no. SNU-120313-10-1). Cell culture C 2 C 12 (mouse mesenchymal precursor), MC3T3-E1 (mouse pre-osteoblast) and HEK293T (human embryonic kidney) cell lines were obtained from American Type Culture Collection (ATCC; Manassas, VA). Cells were cultured at 5% CO 2 in Dulbecco’s modified Eagle's medium, supplemented with 10% heat-inactivated fetal bovine serum. C 2 C 12 differentiation towards osteoblast was induced by BMP-2 (100 ng ml −1 ) or Wnt3a (50 ng ml −1 ). ATDC5 cell line (mouse chondrocyte), which was a kind gift from Dr Dae-Won Kim (Yonsei University, Korea), was cultured at 5% CO 2 in 1:1 mixture of DMEM and Ham’s F-12 medium containing 10% FBS. ATDC5 differentiation was induced by Insulin-Transferrin-Selenium Supplement (Life Technologies) and BMP-2 (10 ng ml −1 ). Critical-size calvarial defects in rats Male Spraque–Dawley rats (10 weeks old) were purchased from Orient Bio Inc (Gyeonggi-do, Korea) and kept in specific pathogen-free rooms. General anaesthesia was induced using Zoletil and Rumpun. After a midline incision of the scalp, an 8-mm critically sized calvarial defect was created using a trephine bur (GEBR; Brasseler, Germany) under sterile saline irrigation. The calvaria was covered with a 1% collagen matrix (Bioland; Cheongwon, Korea) containing BMP-2 (1 mg) and shCon or shNAA10 (5.0 × 10 9 ml −1 ), and skin flaps were sutured. Six rats per each group were killed 6 weeks after surgery. The calvarias were decalcified with 10% EDTA solution for 2 weeks and dehydrated through a series of ethanol solutions of increasing concentration and embedded in paraffin. The calvarial slices (5 μm thickness) were sectioned coronally at the centre of defect, stained with H&E, and subjected to immunohistochemistry. The procedures used and the care of animals were approved by Institiue of Laboratory Animal Resources Seoul National University (approve no. SNU-111111-3) and adhered to the Seoul National University Laboratory Animal Maintenance Manual. NAA10 transgenic mice Transgenic mice overexpressing m NAA10 235 (mouse orthologue of human NAA10 ) were produced by using modified pCAGGS expression vector containing cytomegalovirus enhancer fused to the ubiquitously expressed chicken β-actin promoter. Purified transgenic construct DNA was microinjected into the fertilized eggs collected from the superovulated C57BL/6 females, as previously described [42] . Genotyping was performed by PCR and Southern blot analysis of genomic DNAs obtained from the tails of founder mice at 2 weeks of age. Two different founders (#10 and #15) were bred in the hemizygous state, and transgenic and non-transgenic littermates were assigned into pair-matched groups for all experiments. Mice were fed a chow diet and water ad libitum in the Ewha Laboratory Animal Genomics Centre under specific pathogen-free conditions. Wild-type and NAA10 transgenic mice were killed on postnatal day 3 to examine the extent of bone development. After the skulls were carefully isolated from skin and brain, they were washed with PBS and fixed in 10% formalin for 24 h. All experiments were approved by the Institutional Animal Care and Use Committees of Ewha Women’s University, and adhered to the National Research Council Guidelines (approve no. 2010-24-2). NAA10 -knockout mice Naa10 -knockout mice were generated based on a standard gene-targeting in E14 embryonic stem (ES) cells (129/Sv). The targeting vector was constructed to delete exons 1–4 in the Naa10 gene. ES cells were electroporated with the targeting vector that was linearized with Not I, and selected by neomycin and gancyclovir. Selected clones were screened for homologous recombination using Southern analysis. Correctly targeted ES clones were used for blastocyst microinjection and generation of chimeric mice. Chimeric mice were mated with C57BL/6 mice, and germ-line transmission of targeted alleles was detected by PCR and Southern blot analysis. Naa10 -knockout mice were backcrossed more than 10 times into the C57BL/6J background. Genotyping was performed by PCR and Southern blot analyses of genomic DNAs obtained from the tails. All experiments were performed according to the protocol approved by the Institutional Animal Care and Use Committees (IACUC) of Ewha Women’s University. Histological procedure and histomorphometric analysis Calvaria, tibia and vertebra tissues were decalcified with 10% EDTA solution for 2 weeks and dehydrated through a series of ethanol solutions of increasing concentration and embedded in paraffin. The calvarial slices (5 μm thickness) sectioned coronally were stained with H&E. Digital images of H&E-stained calvaria sections were taken using OLYMPUS microscope and camera (Tokyo, Japan) and the following histomorphometric paramenters were analysed by OsteoMeasure version 1.01 software (Osteometrics, Decatur, GA). Each parameter was analysed in quadruplicate from four different images per H&E-stained section at 400-fold magnification and its mean value was calculated from five independent experiments. The number of osteoblasts per bone perimeter (N.Ob/B.Pm, 1 mm −1 ) and the percentage of osteoblast surface to bone surface (Ob.S/BS, %) were determined according to standardized protocols using the OsteoMeasure programme. Histomorphometric data are presented as recommended by the American Society for Bone and Mineral Research. Micro-CT-based analysis of bone structure Calvarial bones were removed and fixed in 10% formalin, and micro-CT was taken using NFR Polaris-G90 manufactured by Nanofocusray (Jeonju, Korea). The scanner uses an X-ray source and has a camera that rotates around a bed holding the samples. The samples were scanned at a tube potential of 65 kVp and a tube current of 120 μA for 15 min. Data were acquired from the 1,024 images of reconstruction with an isotropic voxel spacing of 0.034 × 0.034 × 0.027 mm 3 . The volume of bone ingrown in a defect site was analysed by the three-dimensional analysis using a software Amira version 5.4.1 (San Diego, CA). The bone range was reflected with CT analyzer manual, which ranged more than 1,000 CT number, and the CT number of air (1,000 HU) and water (0 HU) was used to calibrate the image values in Hounsfield units. To distinguish bone tissue from soft tissue, the CT number was given a range of brain and cortical-bone equivalent hydroxyapatite material. The mean value was determined by the CT number. The bone parameters bone volume/tissue volume (BV/TV, %), bone (for calvaria) or trabecular (for femur) thickness (Tb.Th, mm), bone or trabecular number (Tb.N, 1/mm) and trabecular separation (Tb.Sp, mm) were calculated using the analysis software CTAn v1.9 and the three-dimensional model visualization software μCTVol v2.0. The scanner was set at a voltage of 40 kVp, a current of 200 μA and a resolution of 11.55 μm pixels. The femur sample area selected for scanning was a 1.5-mm length of the secondary spongiosa, originating 1.0 mm below the epiphyseal growth plate. Alcian blue/Alizarin red co-staining of skeletons After the skin and internal organs were removed, mice were fixed in ethanol for 5 days. Mice were stained with 0.015% Alcian Blue 8GX and 0.005% Alizarin Red S in ethanol/acetic acid (9:1. v/v) at 37 °C for 48 h. After being rinsed with water, skeletons were kept in 1% KOH solution with 20% glycerol until they became clearly visible. Alkaline phosphatase, alizalin red S and von Kossa stainings C 2 C 12 cells were cultured on 6-well plates at a density of 1x10 5 cells per well, and ALP was visualized using naphthol AS-MX phosphate (Sigma-Aldrich) as a substrate. After being differentiated by BMP-2, cells were fixed with 10% formaldehyde for 5 min, briefly rinsed by water and permeabilized by 0.1% Triton X-100. Cells were incubated at 37 °C for 30 min in a mixture containing sodium nitrite, FRV-Alkaline solution (Sigma-Aldrich) and Naphthol-AS-BL alkaline solution (Sigma-Aldrich). After being rinsed by water, wells were photographed. The calcification of osteoblast was analysed by Alizarin Red staining. After being fixed in 10% formaldehyde and washed with distilled water, cells were stained with 1% Alizarin Red S at room temperature for 20 min. Wells were rinsed with water and photographed. Mineralization of bone tissues was evaluated by von Kossa staining. Rat calvarias were fixed with 3.7% paraformaldehyde and embedded in epoxy resin. Calvarial sections were incubated with 1% silver nitrate and exposed to bright light for 30 min. After silver was removed by 5% sodium thiosulfate, sections were counterstained with Nuclear Fast Red. ALP activity The cultures were rinsed twice with ice-cold PBS, solubilized in a lysis buffer (pH=10.5, 50 mM Tris, 100 mM glycine and 0.1% Triton X-100) and sonicated twice on ice for 15 s. The supernatant was collected and used to determine total protein and ALP levels. Total protein levels were calculated using a BCA protein assay kit (Bio-Rad; Hercules, CA). A 100-μl aliquot of freshly prepared p -nitrophenyl-phosphate tablet solution was added to 200 μl of the supernatant samples and incubated at 37 °C for 30 min. The optical density of p -nitrophenol was measured at 405 nm, and ALP activity was standardized as nmoles of p -nitrophenol per mg of protein per minute. RT-PCR Total RNAs were extracted using TRIZOL (Invitrogen), and reverse transcribed in a reaction mixture containing M-MLV Reverse Transcriptase (Promega; Madison, WI), RNase inhibitor, dNTP and random primers at 46 °C for 30 min. For sensitive semi-quantitative RT-PCR, the cDNAs were amplified over 17 PCR cycles with 5 μCi [α- 32 P]dCTP. The PCR products were electrophoresed on a 4% polyacrylamide gel, and the dried gel was autoradiographed. PCR primer sequences are 5′-AACCTCAAAGGCTTCTTCTT-3′ and 5′-ACATGGGGAATGTAGTTCTG-3′ for mouse ALP and 5′-AAGAGAGGCATCCTCACCCT-3′ and 5′-ATCTCTTGCTCGAAGTCCAG-3′ for mouse β-actin. Quantitative real-time PCR was performed in the Evagreen qPCR Mastermix, and fluorescence emitting from dye-DNA complex was monitored in CFX Connect Real-Time Cycler (BIO-RAD). The levels of mRNAs were normalized by 18S RNA levels and represented as relative values. The primer sequences are 5′-GCAATAAGGTAGTGAACAGACTCC-3′ and 5′-GTTTGTAGGCGGTCTTCAAGC-3′ for mouse OCN; 5′-AAGCAGCACCGTTGAGTATGG-3′ and 5′-CCTTGTAGTAGCTGTATTCGTCCTC-3′ for mouse BSP; 5′-AACCTCAAAGGCTTCTTCTT-3′ and 5′-ACATGGGGAATGTAGTTCTG-3′ for mouse ALP; 5′-AACTTCTGTGGGAGCGACAA-3′ and 5′-GGGAGGGAAAACAGAGAACGA-3′ for mouse sex determining region Y-box 9 (Sox9). Reporter assays Cells were cotransfected with 6xOSE-luciferase or OG2-luciferase and CMV-β-gal using calcium phosphate or Lipofectamine reagent. The final DNA or siRNA concentration was adjusted by adding pcDNA or control siRNA, respectively. After 16 h of stabilization, transfected cells were seeded on four dishes at a cell density of 5 × 10 4 cells cm −2 and further cultured for 24 h. The cells were incubated under normoxic or BMP-2 treated conditions for 48 h, and then lysed to determine luciferase. β-gal activities were measured to normalize transfection efficiency. Preparation of cytosolic and nuclear extracts Cells were centrifuged at 1,000 g for 5 min, and resuspended with a lysis buffer containing 10 mM Tris/HCl (pH 7.4), 10 mM KCl, 1 mM EDTA, 1.5 mM MgCl 2 , 0.2% NP40, 0.5 mM dithiothreitol, 1 mM sodium orthovanadate and 400 μM phenylmethylsulphonyl fluoride. The cell lysates were separated into pellet (for nuclear fraction) and supernatant (for cytosolic faction) using centrifugation at 1,000 g for 5 min. One packed volume of a nuclear extraction buffer (20 mM Tris/HCl, pH 7.4, 420 mM NaCl, 1 mM EDTA, 1.5 mM MgCl 2 , 20% glycerol, 0.5 mM dithiothreitol, 1 mM sodium orthovanadate, and 400 μM phenylmethylsulphonyl fluoride) was added to the pellet, and vortexed intermittently at low speed on ice for 30 min. The nuclear extracts were cleaned at 20,000 g for 10 min, and stored at −70 °C. Immunoblotting and immunoprecipitation Cell lysates were separated on SDS-polyacrylamide (8–12%) gels, and transferred to an Immobilon-P membrane (Millipore, Bedford, MA). Membranes were blocked with a Tris/saline solution containing 5% skim milk and 0.1% Tween-20 for 1 h and then incubated overnight at 4 °C with a primary antibody diluted 1:1,000 in the blocking solution. Membranes were incubated with a horseradish peroxidase-conjugated secondary antibody (1:5,000) for 1 h at RT, and stained using the ECL-plus kit (Amersham Biosciences, Piscataway, NJ). To analyze protein interactions, cell lysates were incubated with anti-Runx2, anti-Myc or anti-Flag antibody (2 μg ml −1 ) overnight at 4 °C, and the immune complexes were pulled down by 10 μl of protein A/G beads (Santa Cruz, CA). The bound proteins were eluted in a denaturing SDS sample buffer or by Myc/Flag peptides, loaded on SDS–polyacrylamide gel electrophoresis (PAGE) and immunoblotted with anti-Runx2, anti-NAA10, anti-Myc or anti-Flag antibody. Chromatin immunoprecipitation Cells were fixed with 1% formaldehyde for 10 min to crosslink chromatin complexes, and treated with 150 mM glycine to stop the crosslinking reaction. After cells were lysed and sonicated, soluble chromatin complexes were precipitated with anti-Runx2 antibody (10 μg ml −1 ) overnight at 4 °C. DNAs were isolated from the precipitates and the precipitated DNA segment of the OCN promoter was quantified by real-time PCR using the Evagreen qPCR Mastermix (Applied Biological Materials, Inc., Richmond, Canada) in the CFX Connect Real-Time System (BIO-RAD). The chromatin immunoprecipitation-DNAs were amplified over 40 PCR cycles (95–53–70 °C, 20 s at each temperature) and the DNA amplification was continuously monitored. The primer sequences used for qPCR amplifying the OCN gene are 5′-TGCATAGGGTTCTTGTCTCT-3′ and 5′-CTCCACCACTCCTACTGTGT-3′. In vitro acetylation assay GST-tagged Runt domain, its K225R mutant or His-tagged NAA10 peptide was expressed in E. coli using isopropyl-β- D -thiogalactoside, and then purified using GSH- or nickel-affinity beads. Recombinant His-NAA10 (0.5 μg) and GST-Runt (0.5 μg) peptides were incubated in a reaction mixture (50 mM Tris/HCl pH 8.0, 0.1 mM EDTA, 1 mM DTT, 10 mM sodium butyrate, 20 mM acetyl-CoA and 10% glycerol) at 37 °C for 4 h. Acetylated Runt peptides were identified by western blotting using anti-acetyl lysine antibody. To verify the presence of peptides, the mixture was run on a SDS-polyacrylamide gel and stained with 0.1% Coomassie Brilliant Blue R-250, followed by being destained with 50% methanol and 10% glacial acetic acid. In-gel digestion and mass spectrometric analysis After F/S-Runt peptide was coexpressed with NAA10 in C 2 C 12 , the peptide was separated by a SDS–PAGE, digested in the gel slice with trypsin and subjected to a nanoflow ultra-performance liquid chromatography/ESI/MS/MS with a mass spectrometer (Q-tof Ultra global), comprising a three-pumping Waters nano-liquid chromatography system, a stream selection module and MassLynx 4.0 controller (Waters, UK). Five microlitres of mixed peptides was dissolved in buffer C (water/acrylonitrile/formic acid; 95:5:0.2, V:V:V), injected on a column and eluted by a linear gradient of 5–80% buffer B (water/acrylonitrile/formic acid, 5:95:0.2) over 120 min. MS/MS spectra were processed and analysed using ProteinLynx Global Server (PLGS) 2.1 software (Micromass, UK). Lysyl acetylation was identified by the additional mass of 42 Da on lysine residue. Antibody generation Antibody against acetylated K225 of Runx2 was raised from rabbits (New Zealand white). Rabbits were immunized with Keyhole limpet haemocyanin-conjugated synthetic peptide ( Supplementary Fig. 22a ), which contain acetylated K225 of Runt domain in Runx2. The specific, polyclonal antibody was purified by affinity chromatography using the acetylated K225 peptide. Statistics All data were analysed using Microsoft Excel 2007 software, and results are expressed as means and s.d. We used the unpaired, two-sided Student’s t -test to compare reporter activities and morphometric data from micro-CT analyses. Statistical significances were considered when P values were less than 0.05. How to cite this article : Yoon, H. et al. NAA10 controls osteoblast differentiation and bone formation as a feedback regulator of Runx2. Nat. Commun. 5:5176 doi: 10.1038/ncomms6176 (2014).